The intriguing dual-directing effect of 2-cyanobenzyl ether for a highly stereospecific glycosylation reaction The diverse presence as well as their very specific bio-responses of glycoconjugates found in all living species requires scientists to synthesize the precise structure of these complex oligosaccharides for various studies on glycoscience. Very few approaches were able to offer the sole α- or β-glycosylated products, even at the cost of complicating the preparative route or usage of exotic chiral auxiliaries to drive the stereoselectivity. In this report, the unification of solvent assistance and neighbouring group participation concepts have led us to the use of 2-cyanobenzyl ether as the dual-directing auxiliary for stereospecific construction of α- and β-glycosidic bonds from a single starting material, and both isomers can be obtained in exclusive stereoselectivity. This work demonstrates the difference in reactivities of glycosyl acceptors can be employed to completely drive the stereoselectivity, drawing the parallel comparison with the arming/disarming concept, which has been exclusively confined to glycosyl donors. The ubiquitous presence of carbohydrate structures on all cell surfaces and interstitial space has been recognized as playing vital roles in the development and communication of living organisms [1] , [2] . Studies of such important macromolecules were often hampered by the inherent diversity in composition as well as stereochemistry of glycosidic bonds. While recent approaches [3] , [4] have greatly improved our ability to control the stereooutcome of glycosylation reactions, an efficient and universal method is still highly sought after, especially one that is applicable for large-scale as well as combinatorial chemistry. One of the earliest and yet very effective way to acquire the desired anomeric stereoselectivity was through employment of participating solvents, notably nitrile-type [5] , [6] (for example, acetonitrile) or ether-type [7] (for example, diethyl ether) for the preferential formation of β- D - and α- D -glucosides, respectively. On the other hand, neighbouring hydroxyl groups of the donor could show influence on the anomeric preference through their protecting substituents, many of which were routinely exploited in various glycosylation methods, such as 2 -O -ester-type [8] , [9] , [10] or 2 -O -picolyl-type [11] , [12] , [13] for 1,2- trans glycosylation, and several sulfide auxiliaries [14] , [15] , [16] , [17] , [18] as well as intramolecular aglycon delivery IAD-type [19] , [20] for 1,2- cis glycosylation reactions. We envisage that a combination of these two directions could deliver an attractive solution to construct most types of glycosidic bonds, with the potential to overcome current drawbacks. Herein, we demonstrate a highly stereoselective glycosylation method through 2-cyanobenzyl ether functionalization at C-2 position of various glycosyl donors. The results come with a surprising twist: from a single glycosyl donor, either α- or β-glycosylated products can be predicted and obtained through modification of the glycosyl acceptors. Compatibility with a wide collection of protective choice, leaving groups and versatile activations under acidic or basic conditions highlight the potential of 2-cyanobenzyl ether as the universal auxiliary for glycosylation reactions. Design and optimize the conditions First, we studied a glycosyl donor bearing a solvent-like moiety. An ether- or nitrile- group was attached to the glucosyl donor through an optimal scaffold, which was chosen to be benzyl ether-type due to its stability and routine use in carbohydrate syntheses. Assessment of literature reports for this kind of structure led us to the concept of arming participating groups [11] , [12] , [13] , hitherto materialized in the use of 2 -O -picolyl [11] , [12] , [13] and most recently 2 -O -nitrobenzyl [21] ether. Preliminary results showed virtually no directing effect of 2-methylthiobenzyl ether 1a ( Fig. 1a ), similar to the 2-methoxybenzyl ethers in the previous study [11] . In contrast to the use of chiral six-membered sulfide by Boons et al . [14] , [15] , which favoured the trans -decalin sulfonium intermediate, our hypothetical seven-membered intermediate should give more flexibility to overwhelm the β-prefered [14] , [15] , [16] , [17] , [18] coordination of the sulfide. 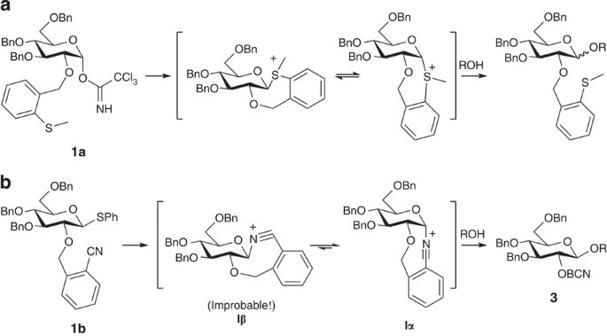Figure 1: Solvent-like participating groups and their theoretical intermediates. (a) Glycosylation with 2-methylthiobenzyl ether at C-2. (b) Glycosylation with 2-cyanobenzyl ether (BCN) at C-2. Figure 1: Solvent-like participating groups and their theoretical intermediates. ( a ) Glycosylation with 2-methylthiobenzyl ether at C-2. ( b ) Glycosylation with 2-cyanobenzyl ether (BCN) at C-2. Full size image Henceforth, we decided to focus on the 2-cyanobenzyl ether [22] , [23] , [24] 1b ( Fig. 1a , abbreviated as BCN), from an intuitive conjecture that nitrile solvents were found computationally and experimentally to form the nitrilium ion with α-exclusivity [25] , [26] , [27] . Second, the linear nature of nitrile would prevent β-coordination due to significant bond-angle strain. Our theoretical calculation substantiated this proposal: conformation Iα is more energetically favoured than β-coordinated Iβ , by a difference of 13.37 kJ mol −1 ( Supplementary Fig. 53 , DFT, B3LYP/6-31+G(d) level). Both species were found to be more energetically favoured than the non-coordinated oxocarbenium ion. Optimizing experiments were first conducted with common activating conditions, such as NIS/AgOTf, NIS/TMSOTf and Ph 2 SO/Tf 2 O/TTBP ( Table 1 , entries 1–4). Initial results indicated very low selectivity under ice-bath cooling. Lowering temperature to −60 °C significantly elevated stereoselectivity to over 10β:1α ( Table 1 , entry 5). Further decrease to −78 °C upon the addition of n -butanol improved the yield as well as the selectivity ( Table 1 , entry 6). A survey of various solvents revealed that toluene can provide the optically pure β- 3b ( Table 1 , entry 7), amidst CH 2 Cl 2 , THF, Et 2 O, EtCN. Within nuclear magnetic resonance (NMR)-limited sensitivity the α-product was undetectable. This β-product was found to be the major isomer in all solvents, even under α-promoting media ( Table 1 , entries 8 and 9). No chemical conversion was observed when propionitrile was used, and all starting materials were recovered ( Table 1 , entry 10). Table 1 Optimization studies. Full size table In general, the structure of glycosyl acceptors only shows complementary effects [28] on stereoselectivity of a glycosylation reaction, compared with the structure of donors [29] , [30] , [31] , and other factors such as temperature or solvents. Glycosyl acceptors bearing electron-withdrawing substituents should diminish the nucleophilicity of the hydroxyl group, resulting in a decrease of reaction rate [29] , [32] . This could improve selectivity as the reaction can be carried out in a more controlled manner [33] . However, we were surprised to observe a complete reversal of anomeric preference when TFE (2,2,2-trifluoroethanol) was used as the acceptor. Under β-optimized condition, α- 3h was obtained as the major product with an α:β ratio of >17:1 ( Table 1 , entry 12). Re-examination of solvents returned α- 3h as the sole isomer when diethyl ether was used ( Table 1 , entry 14). Within NMR-limited sensitivity the β-product was undetectable. Nonetheless, a striking difference between butanol and TFE is very apparent, which could not be satisfyingly explained with the anomeric effect [34] and/or solvent influence [5] , [6] , [7] . Expand the substrate scopes From these optimized conditions, we made a tentative suggestion that pure β-anomers would typically be obtained, whereas sole α-anomers were produced with glycosyl acceptors with electron-withdrawing functional groups. Subsequently, evaluation on the versatility of this reaction was carried out by studying a diversified substrate scope. 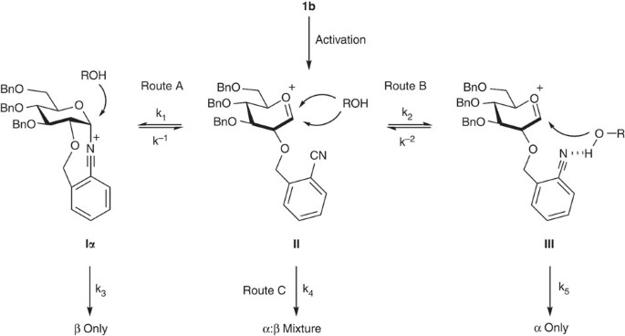Figure 2: Proposed mechanism for the dual-directing effect of 2-cyanobenzyl ether. (Route A) β-only pathway through SN2 displacement of nitriliumIα.(Route B)α-only pathway through H-bond-assisted glycosylation ofIII.(Route C)α:β mixture pathway through oxocarbenium ionII. As seen from Table 2 , reaction of various common alcohols, including n -butanol 2b , benzyl alcohol 2c , 1-adamantanol 2d proceeded smoothly to give glycosylated products with β-only stereoselectivity. More bulky and complex alcohols, such as citronellol 2e , fenchol 2f and cholesterol 2g all gave desired products in good yields. With the exception of 2,2,2-trifluoroethyl-α- D -glucopyranoside 3h giving α-product so far, we proceeded to prepare acceptors for disaccharide surveys. For each hydroxyl group position, pair of acceptors having electron-donating or electron-withdrawing protective groups were synthesized. To our delight, the results substantiated our earlier prediction of the correlation between stereoselectivity and acceptor structure ( 2i , 2j , 2k for 2-OH; 2l , 2m , 2n for 3-OH; 2o , 2p for 6-OH). However, with acceptors 2s and 2t for 4-OH position, reactions were extremely sluggish under optimized conditions. The well-known unreactive nature of 4-OH was suggested previously to emerge from steric crowding [24] , [35] , [36] . Accordingly, various improvements have been documented, including introduction of a cyclic N -acetyloxazolidinone [35] , [36] or 1,6-anhydropyranoside with an inverted 1 C 4 conformation [37] to enhance performance. Gratifyingly, the acceptor 1,6:2,3-dianhydro-β- D -mannopyranose 2q proceeded smoothly to provide 3q with exclusive β-1,4 linkage. Since this acceptor is electron rich, we decided to introduce the azido at C-2 and benzoyl at C-3 of acceptor 2r as electron-deficient groups. As expected, we obtained the α-1,4-linked disaccharide 3r in 81% yields. 1,6-anhydro pyranosides [38] are very versatile and useful scaffolds to construct functionalized 1,4-glycosides and 1,4-glycosamines as well. Having successfully synthesized both α- and β-products with hydroxyl groups at every position, we turned our attention to evaluate different protecting groups on glucosyl donors and different sugar donors. Exclusive selectivities of 3b and 3h were again obtained with 1c bearing trichloroimidate as the leaving group. Per-acetylated donor 4a was similarly activated with catalytic TMSOTf to deliver β- 5a and α- 5b anomers in excellent yields. However, because the acidic environment was found detrimental to the acid-labile 3,4 -O -isopropylidene group on galactoside 6b , its precursor 6a was directly activated instead under an identical condition to 1b to give β- 7a and α- 7b . Table 2 Exploration of substrate scopes. Full size table A plausible mechanism to explain dual-directing outcome in stereoselectivity is depicted in Fig. 2 . Activation of 1b forms oxocarbenium ion II , which exists in equilibrium with nitrilium ion Iα , resulting from the solvent-like coordination of the nitrile moiety to the anomeric carbocation. Direct glycosylation of acceptor with intermediate II via route C would produce a mixture of isomers, whereas displacement of nitrilium through route A would afford the β-isomer since the axial position was thoroughly occupied. Although this equilibrium could justify the β-exclusivity for a majority of substrates, it was insufficient to account for the complete reversal to α-stereoselectivity with selected acceptors. A careful structural analysis of both donor and acceptors lead us to include route B, in which the active donor species was oxocarbenium ion II . The incipient acceptor could form hydrogen bonding [39] , [40] with the nitrile [41] functional group (via intermediate III ). Preceding any direct glycosylation, the acceptor would be driven to target the anomeric carbocation from an axial trajectory to generate the 1,2- cis product. Figure 2: Proposed mechanism for the dual-directing effect of 2-cyanobenzyl ether. (Route A) β-only pathway through S N 2 displacement of nitrilium Iα . (Route B) α-only pathway through H-bond-assisted glycosylation of III . (Route C) α:β mixture pathway through oxocarbenium ion II . Full size image Our rationale derived from the arming nature of the glycosyl donor: there is less destabilization with tetra -O -benzyl ethers on oxocarbenium ion II , thus allowing facile equilibrium shift between the three active species. Second, considering the nitrile group to be a weak H-acceptor, it is reasonable that sufficient H-bonding can only occur to stronger H-donors [42] . Incidentally, electron-poor alcohols not only increased donoring ability of the proton, but also decreased nucleophilicity on the oxygen atom [43] . Consequently, glycosylations through routes A and C would be suppressed while H-bond-assisted glycosylation through route B would remain less affected since the nucleophile was brought closer to the reaction centre. Third, H-bonding interaction could be active from a more distant start and requires lesser activation energies [44] , [45] than formation of a covalent bond in other routes. Counter-wise, the weak H-bonding with usual acceptors would be of minor influence, making route A the dominant course. Experimental evidence support the proposed hypothesis as well as provide deeper insights into the mechanism (see supporting information for the results). Trapping experiments were found to give cyclic α-imidate 3u and α-imide 3v when the glycosyl acceptor was 2-chlorobenzoic acid ( Fig. 3 ). The peculiar value of anomeric coupling ( δH =5.87, J 1,2 =7.6 Hz) correlates well with original report probing the nitrile effect on acetontrile [25] , [26] , [27] ( δH =5.97, J 1,2 =7.3 Hz). This resulted from the substantial flattening of pyranose ring at C-1 and C-2 due to steric bulk of imide. The absence of any β-imide 3v produced validated route A mechanism with complete α-coordination of the nitrile. One-dimensional (1D) selective TOtal Correlated SpectroscopY (TOCSY) experiments were conducted to individually reveal NMR chemical shifts of 3u and 3v (see Supplementary Methods ). 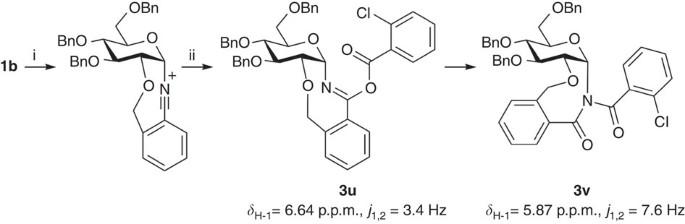Figure 3: Trapping experiment with 2-chlorobenzoic acid25,26,27. Reaction conditions: (i) Ph2SO, Tf2O, TTBP, −60 °C. (ii) 2-ClC6H4CO2H, −78 °C. Figure 3: Trapping experiment with 2-chlorobenzoic acid [25] , [26] , [27] . Reaction conditions: ( i ) Ph 2 SO, Tf 2 O, TTBP, −60 °C. ( ii ) 2-ClC 6 H 4 CO 2 H, −78 °C. Full size image Several lines of evidence validated α-directing glycosylation through coordination between acceptor and the BCN group. First, based on insightful studies by Vasella [46] , [47] and Crich [24] , our detailed H-bond NMR study showed negligible interaction between ethanol and 1b but showed notable chemical shifts of OH when electron-poor TFE was mixed with 1b ( Supplementary Figs 45 and 46 ). Second, competitive reactions were conducted to verify the arming nature of 2-cyanobenzyl ethers as well as provide more credence to α-directing effect: an equimolar amount of compound 1b was mixed with phenyl 2,3,4,6-tetra- O -benzyl-β- D -thioglucoside 1w . Following activation of the donors under optimized conditions, an equivalent of n -butanol was subsequently introduced ( Fig. 4 ). Two butylglucosides were obtained as expected, with comparable yields. This showcased that the nitrile functional group had minimal influence on the arming of benzyl ether linkage. More importantly, excellent stereoselectivity was obtained only with the BCN auxiliary, whereas the non-participating 1w gave in a mixture of isomers (5.5β:α). 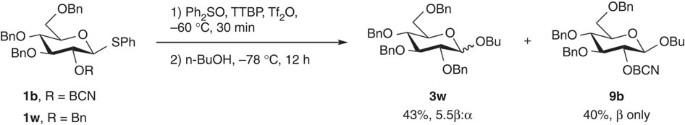Figure 4: Competitive reaction between two arming donors. SeeSupplementary Methodsfor complete results of the competitive reactions and the possible role of triflate ions. Figure 4: Competitive reaction between two arming donors. See Supplementary Methods for complete results of the competitive reactions and the possible role of triflate ions. Full size image On the basis of very insightful studies by Demchenko et al . [11] , [12] , [13] on proving the existence of H-bonding between an auxiliary-equipped donor and acceptor, a survey of effects that could reduce stereoselectivity by disrupting the H-bonding was examined in Table 3 . Table 3 A survey of effects that disrupt H-bonding. Full size table For this mechanistic study, we used dichloromethane as the non-participating solvent. When electron-rich acceptor 2o was added at 0 °C, mixture of 3o was obtained (entry 1), indicating no selectivity. This stood in stark contrast to 2p , which gave in a 7α:1β mixture of 3p (entry 2). Should non-stereoselective pathway (via II , Fig. 3 ) or solvent choice solely be responsible for the anomeric ratio, we should observed donor 1c giving a similar result to entry 1 and 2,3,4,6-tetra- O -benzyl donor from other reports [48] , [49] . Also consistent with the known phenomemnon that H-bond can be disturbed by addition of dimethyl sulfoxide, introduction of this species led to decrease in stereoselectivity (entry 3). As suggested in a previous report [12] , the possible role of glycosyl sulfoxonium ion remained speculative and may not have significant effect. Third, the use of the trimethylsilane (TMS)-protected counterpart of glycosyl acceptors 2o as 2o* and 2p as 2p* led to very different results: 2o* gave very low yield and selectivity of 3o (entry 4) while 2p* still furnished 3p in excellent α:β ratio (entries 5 and 6). The result indicated that trimethylsilyl can act as a proton-like moiety to interact with BCN auxiliary, but this is only possible with electron-withdrawing nucleophiles such as 2p* . There were reports on weakly basic solvents [50] , [51] such as acetonitrile or toluene that were capable of forming isolated species of the type R3Si(solvent)+, reflecting the extraordinary electrophilicity of the silylium cation [52] , [53] . On the other hand, stereoselectivity was significantly degraded when an excess amount of TMSOTf (entry 7) or HOTf (entry 8) was added. The presence of these electrophilic species in ample quantities likely disrupts the mechanism, deteriorating the stereoselectivity. In addition, to affirm the presence of I , the activation of 1b was conducted in deuterated toluene-d8 at −60 °C. However, immediately after addition of Tf 2 O, the solution quickly darkened and a brown solid was precipitated. The resulting heterogenous mixture prevented us from obtaining 1 H-NMR, whereas 13 C-NMR showed disappearance of any carbohydrate species. The inclusion of many active reagents in excess could be responsible for the incident. Switching the solvent to CD 2 Cl 2 gave a very complicated spectra, which was due to benzylic protons obscuring important chemical shifts. Hence, we decided to use donor 4a and catalytic amount of TMSOTf as the activator for the low-temperature NMR study. From Fig. 5 , addition of TMSOTf to the NMR tube at −78 °C in a dry-ice Delaware flask, followed by quickly transferring it to the NMR spectrometer (method A) led to partial activation of 4a and the presence of two new glucosyl species: the α-nitrilium glucoside IV (H-1 was a doublet at 6.36 p.p.m. with J =2.4 Hz, C-1 at 104.3 p.p.m.) and N -trichloroacetylglucosylamines V ( H-1 was a doublet of doublet at 5.88 p.p.m. with J =6.8 Hz, 2.8 Hz, C-1 at 76.2 p.p.m.). V was the product of the acid-catalysed rearrangement of anomeric trichloroacetimidate [54] . After 10 min, 4a was completely consumed and the ratio of IV : V remained constant at 1:1.15 after 1 h, with no observed interconversion or decomposition. 1D-TOCSY and HSQC (see Supplementary Methods ) were conducted to individually reveal the chemical shifts of each species and no other glucosyl intermediates, including β-coordinated nitrilium or glucosyl triflates, were detected. To suppress the formation of V , in method B, the NMR tube containing 4a was put in NMR spectrometer for 15 min and was briefly lifted up to inject TMSOTf, and immediately put back into the NMR probe. The ratio of IV:V was >20:1 and remained constant at −78 °C. 13 C-NMR of IV was recorded and compared with 4a and mixture of IV : V in method A. As the temperature increased, the nitrilium IV was slowly converted to glucosylamine V . Above −10 °C, IV was thoroughly consumed in a matter of few minutes. All the results substantiated there was preference for anomeric nitrilium IV at very low temperature and confirmed the nitrile groups were responsible for the dual-stereoselective glycosylation. 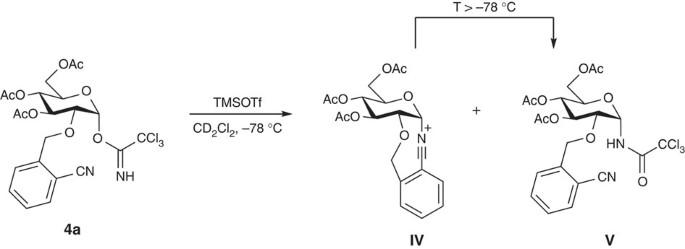Figure 5: Low-temperature NMR study. It is noteworthy that concentration of intermediateIVremained unchanged at −78 °C and no anomeric triflate was observed. Figure 5: Low-temperature NMR study. It is noteworthy that concentration of intermediate IV remained unchanged at −78 °C and no anomeric triflate was observed. Full size image Finally, removal of BCN ether was no different from the usual benzyl ethers, as shown in the deprotection of 3b to give the n -butyl-β- D -glucopyranoside 8b ( Fig. 6 ). THF was found to offer excellent conversion compared with methanol or ethyl acetate. 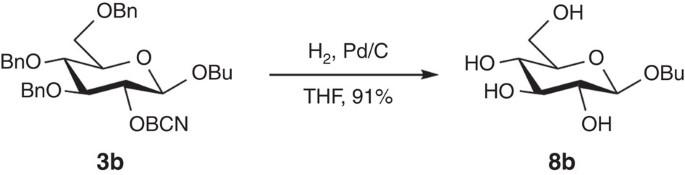Figure 6: Removal of the 2-cyanobenzyl ether. It is noteworthy that THF was found to be superior to methanol or ethyl acetate. SeeSupplementary Methodsfor the deprotection of compound3b. Figure 6: Removal of the 2-cyanobenzyl ether. It is noteworthy that THF was found to be superior to methanol or ethyl acetate. See Supplementary Methods for the deprotection of compound 3b . Full size image In conclusion, we report an efficient and highly stereospecific glycosylation reaction utilizing BCN ether as a versatile directing group, capable of providing exclusive α-/β-anomers via rational selection of glycosyl acceptors, meanwhile using a single type of donor. The ease of installation, removal (see Supplementary Methods ), robust stability and the precise dual-stereospecificity, which BCN ether could offer, makes it an excellent universal donor for complex carbohydrate syntheses. Future work on mechanistic study as well as refining the method for preparation of various glycoconjugates are in progress. General The synthesis and characterization of new compounds are provided in the Supplementary Methods . For NMR analysis of the compounds in this article, see Supplementary Figs 1–52 . For computational results and atom coordinates, see Supplementary Fig. 53 and Supplementary Discussions . For competitive reactions analysis, see Supplementary Fig. 54 . For H-bonding NMR study, see Supplementary Figs 45 and 46 and Supplementary Discussions . For low-temperature NMR study, see Supplementary Figs 47–52 and Supplementary Discussions . Experimental procedure All reactions were conducted under an atmosphere of nitrogen, unless otherwise indicated. Anhydrous solvents were transferred via an oven-dried syringe. Flasks were flame-dried and cooled under a stream of nitrogen. All reagents and solvents were obtained from commercial suppliers and used without further purification, unless otherwise stated. Chromatograms were visualized by fluorescence quenching with ultraviolet light at 254 nm or by staining using a basic solution of potassium permanganate. Evaporation of organic solutions was achieved by rotary evaporation with a water bath temperature <40 °C. Product purification by flash column chromatography was accomplished using silica gel 60 (0.010–0.063 mm). Technical grade solvents were used for chromatography and distilled before use. Optical rotations were measured in CHCl 3 with a 1-cm cell (c given in g 100 ml −1 ). Melting points were obtained in open capillary tubes in a melting point apparatus. Infrared spectra were recorded using fourier transform infrared spectroscopy and reported in cm −1 . High-resolution mass spectra were recorded on a quadrupole-time-of-flight mass spectrometer. Accurate masses are reported for the molecular ion [M+H] + or a suitable fragment ion. NMR spectra were recorded at room temperature on a 400- and 500-MHz NMR spectrometer. The residual solvent signals were taken as the reference (7.26 p.p.m. for 1 H-NMR spectroscopy and 77.23 p.p.m. for 13 C-NMR spectroscopy). Chemical shifts are reported in delta ( δ ) units, parts per million (p.p.m.) downfield from TMS. Chemical shift ( δ ) is referred in terms of p.p.m., coupling constants ( J ) are given in Hz. Following abbreviations classify the multiplicity: s=singlet, d=doublet, dd=doublet of doublet, t=triplet, q =quartet, m=multiplet, br=broad or unresolved. Assignments were based on analysis of coupling constants and COSY, ROESY, HSQC, 1D-selective TOCSY spectra. Synthesis of compound 3b from 1b Exemplary, a magnetically stirred solution of compound 1b (66 mg, 0.1 mmol), diphenyl sulfoxide Ph 2 SO (28 mg, 0.14 mmol) and 2,4,6-tri-tert-butylpyrimidine (TTBP) (75 mg, 0.3 mmol) in anhydrous toluene (5 ml) was added dropwise triflic anhydride (28 μl, 0.28 mmol, 1 M in CH 2 Cl 2 ) at −60 °C and the temperature was decreased to −78 °C. After 30 min, n -butanol (12 μl, 0.13 mmol) 2b was added dropwise and complete consumption of starting materials was observed after 12 h. Reaction mixture was quenched with triethylamine (0.2 ml) and concentrated under reduced pressure, after which crude NMR was collected, followed by flash chromatography on silica gel to afford compound 3b (55 mg, 90% yield) as a colourless oil. Synthesis of compound 3b from 1c Exemplary, a magnetically stirred solution of n -butanol (12 μl, 0.13 mmol) and 1c (0.71 mg, 0.1 mmol) in anhydrous toluene at −78 °C was added TMSOTf (18 μl, 0.01 mmol). Reaction progress followed by thin-layer chromatography indicates completion of 1c after 12 h. Triethylamine (0.1 ml) was added directly at −78 °C and the temperature was raised to 25 °C. Excess solvent was removed under reduced pressure, after which the crude product was purified with flash chromatography on silica gel to afford compound 3b (51 mg, 83% yield) as a colourless oil. How to cite this article : Le Mai Hoang, K. and Liu, X.-W. The intriguing dual-directing effect of 2-cyanobenzyl ether for a highly stereospecific glycosylation reaction. Nat. Commun. 5:5051 doi: 10.1038/ncomms6051 (2014).